An experimental limit on the charge of antihydrogen The properties of antihydrogen are expected to be identical to those of hydrogen, and any differences would constitute a profound challenge to the fundamental theories of physics. The most commonly discussed antiatom-based tests of these theories are searches for antihydrogen-hydrogen spectral differences (tests of CPT (charge-parity-time) invariance) or gravitational differences (tests of the weak equivalence principle). Here we, the ALPHA Collaboration, report a different and somewhat unusual test of CPT and of quantum anomaly cancellation. A retrospective analysis of the influence of electric fields on antihydrogen atoms released from the ALPHA trap finds a mean axial deflection of 4.1±3.4 mm for an average axial electric field of 0.51 V mm −1 . Combined with extensive numerical modelling, this measurement leads to a bound on the charge Qe of antihydrogen of Q =(−1.3±1.1±0.4) × 10 −8 . Here, e is the unit charge, and the errors are from statistics and systematic effects. The recent creation [1] , [2] , [3] and trapping [4] , [5] , [6] , [7] of antihydrogen has opened new opportunities to explore nature’s fundamental symmetries. The two most often proposed symmetry tests explore CPT (charge-parity-time) invariance by comparing the spectra of antihydrogen with that of hydrogen and probe the weak equivalence principle by measuring the gravitational behaviour of antihydrogen. Recently, the ALPHA collaboration reported initial experimental results in both these areas [8] , [9] ; future experiments expect to obtain much more precise results [9] , [10] , [11] , [12] , [13] , [14] , [15] . Here, we report on a retrospective search for an electric field-induced deflection of antihydrogen atoms as they are released from the ALPHA trap. This search tests for the charge neutrality of these antiatoms, as the antiatoms would only be deflected if they possessed a charge. Theoretically, charge neutrality of antimatter atoms, as well as of matter atoms, is expected from the condition for quantum anomaly cancellation, which is required for theoretical consistency in quantum field theory [16] . Furthermore, experiments show that normal matter atoms and molecules are charge neutral [17] to about 10 −21 e for diverse species such as He, H 2 and SF 6 , where e is the elementary charge. (There do not appear to be precision measurements for H.) As CPT invariance requires that antihydrogen and hydrogen have opposite charge, it predicts that antimatter atoms are charge neutral to a similar level. However, the methods [17] used to test for charge neutrality in normal-matter studies are unsuitable for antihydrogen as they require macroscopic quantities of atoms or molecules; to date, only ~500 antihydrogen atoms have been trapped and detected, and there are no prospects for trapping macroscopic quantities. Thus, an electric field-based deflection measurement of antihydrogen’s charge constitutes a novel test of the fundamental consistencies of quantum field theory and of CPT invariance. We observe a mean axial deflection of 4.1±3.4 mm for antiatoms subjected to an average axial electric field of 0.51 V mm −1 . By using extensive numeric simulations to estimate the mean deflection of putatively charged antihydrogen atoms by these electric fields, as well as those deflections that might be caused by systematic effects, we deduce a bound on the charge of antihydrogen; we find that antihydrogen is charge neutral to Q =(−1.3±1.1±0.4) × 10 −8 (1 σ confidence level), where Qe is the antihydrogen charge, and where the first error is from statistics and the second from known systematic effects. (We note that at the 90% confidence level, the statistical error is ±1.8 × 10 −8 and covers zero.) This bound on the charge of antihydrogen is ~10 6 times lower than the best previous experimental bound [18] . Apparatus and procedures ALPHA traps antihydrogen atoms by producing and capturing them in a minimum-B trap [19] . The trap confines those antiatoms whose magnetic moment is aligned such that they are attracted to the minimum of the trap magnetic field B , and whose kinetic energy is below the trap well depth, . In ALPHA (see Fig. 1a ), this magnetic minimum is created by an octupole magnet, which produces transverse fields of magnitude 1.54 T at the trap wall ( R Wall =22.3 mm), and two mirror coils, which produce axial fields of 1 T at their centres. The mirror coil centres are located at distances z = ±137 mm from the trap centre at z =0 (see Fig. 1b ). These fields are superimposed on a uniform axial field of 1 T produced by an external solenoid [20] , [21] . Taken together, these fields result in an antiatom trap depth of 540 mK, where kelvin is used as an energy unit. 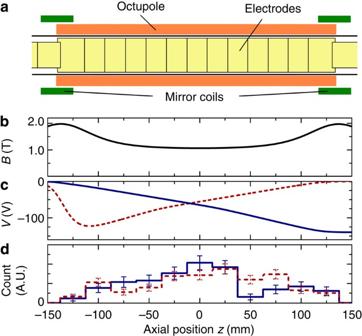Figure 1: Experimental summary. (a) A schematic of the antihydrogen production and trapping region of the ALPHA apparatus, showing the cryogenically cooled cylindrical Penning–Malmberg trap electrodes, and the mirror and octupole magnet coils. Our positron source (not shown) is towards the right, and the antiproton decelerator (not shown) is towards the left. (b) The on-axis magnetic fieldBas a function ofz. (c) The on-axis electrostatic potentialsVused to establish the Bias-Right (red dashed line) and Bias-Left (blue solid line) configurations. (d) Normalized histograms of the experimentalzpositions of the annihilations in the Bias-Right (red dashed line) and Bias-Left (blue solid line) configurations. The error bars show the expected deviation of the distribution based on the number of observed antiatoms in each bin. Figure 1: Experimental summary. ( a ) A schematic of the antihydrogen production and trapping region of the ALPHA apparatus, showing the cryogenically cooled cylindrical Penning–Malmberg trap electrodes, and the mirror and octupole magnet coils. Our positron source (not shown) is towards the right, and the antiproton decelerator (not shown) is towards the left. ( b ) The on-axis magnetic field B as a function of z . ( c ) The on-axis electrostatic potentials V used to establish the Bias-Right (red dashed line) and Bias-Left (blue solid line) configurations. ( d ) Normalized histograms of the experimental z positions of the annihilations in the Bias-Right (red dashed line) and Bias-Left (blue solid line) configurations. The error bars show the expected deviation of the distribution based on the number of observed antiatoms in each bin. Full size image The general methods by which antiatoms are produced from antiprotons and positrons and then captured in our trap are described in refs 4 , 5 , 6 , 22 , 23 , 9 , 10 , 11 , 12 , 13 , 14 , 15 , 16 , 17 , 18 , 19 , 20 , 21 , 22 , 23 . In this Article, we concentrate only on the last phase of the experiments, during which antiatoms are released from the minimum-B trap by turning off the octupole and mirror fields after at least 0.4 s of confinement. The magnet turnoff time constants of ~9 ms result in all antiatoms escaping within 30 ms. The escaping antiatoms are then detected when they annihilate on the trap wall; a silicon-based annihilation vertex imaging detector [24] records the times and locations of the pions that result from the antiproton components of these annihilations. The locations have an axial uncertainty FWHM of 5.6 mm. An electric field, (see Fig. 1c for the corresponding potential), is present in the trap when the antiatoms are released. This electric field would discriminate between antihydrogen atoms and any antiprotons inadvertently left in the trap, as the negatively charged antiprotons would be swept out of the axial ends of the trap [4] , [5] , [25] . As expected [25] , we did not find evidence for any such antiprotons; the application of these electric fields was precautionary. It is these electric fields, however, that allow us to place a bound on the charge of antihydrogen. Two electric field configurations were employed: a Bias-Right (R) configuration, which would sweep antiprotons to the right (positive axial position z ), and a Bias-Left (L) configuration, which would sweep antiprotons to the left (negative z ). Observations In the ~1,300 trapping trials analysed here, 386 of the events recorded by our detector were identified as antiatoms that passed all our selection criteria; these selection ‘cuts’ were determined in ‘blind analysis,’ that is, without reference to the experimental data, and are described in the Methods section below. Of these, 241 were detected in the Bias-Right configuration, and 145 were detected in the Bias-Left configuration. Histograms of their z positions are shown in Fig. 1d , and their average positions are ‹ z › R =7.9±4.2 mm, and ‹ z › L =−0.2±5.3 mm. (The errors associated with these quantities are standard errors of the mean.) These yield sum and difference positions of ‹ z ›=0.5[‹ z › R +‹ z › L ]=3.9±3.4 mm and ‹ z › Δ =0.5[‹ z › R −‹ z › L ]=4.1±3.4 mm, where the errors are found by taking half the quadrature sum of the errors of ‹ z › R and ‹ z › L . The value of the sum ‹ z › is determined by systematic errors discussed in the Methods. A nonzero value for the difference ‹ z › Δ , beyond deviations that could be caused be sampling errors, could only result from a nonzero antiatom charge as there is no other property of the orbital dynamics of the antiatoms that depends on an electric field (aside from a negligible contribution from the polarization of ground state antihydrogen: see Methods). Charge calculation Including the presence of a putative, nonzero charge Q , the on-axis potential energy of an antiatom in the trap is given by where U ( z ) is given using kelvin as an energy unit, is the normalized antihydrogen magnetic moment, verified experimentally in ref. 8 to the accuracy necessary here and k B is the Boltzmann constant. We approximate the electric field inside the trap as the constant E . When Q =0, this potential has a minimum at z =0. Consequently, as B is reduced during the magnet shutdown, the antihydrogen annihilations will be centred around z =0. A nonzero Q will shift the potential minimum, and, hence, the annihilation centre. From equation (1), we can solve for the approximate shift in the minimum of the potential U ( z ) that results from a nonzero Q , or, alternately, the Q required to produce a given size shift ‹ z › Δ , given the average Bias-Right and Bias-Left electric fields, E R and E L , evaluated near the trap centre: Here, we have approximated the quasi-parabolic central magnetic field at the start of the magnet shutdown as B ( z )= B 0 + βz 2 . For our experimental parameters, β =1.6 × 10 −5 T mm −2 , E R =−0.50 V mm −1 and E L =0.52 V mm −1 ; thus, equation (2) predicts Q =−3.7 × 10 −9 (mm −1 )‹ z › Δ . Using the measured ‹ z › Δ yields the approximate Q =(−1.5±1.3) × 10 −8 , where the uncertainty comes from the statistical uncertainty in ‹ z › Δ . While equation (2) allows us to estimate Q , the antiatom orbits in the three-dimensional, time-dependent, fields E and B are sufficiently complicated that numerical simulations [13] , [25] are required to determine the true relation between Q and ‹ z › Δ . Simulations were performed for the Bias-Right and Bias-Left electric fields of Fig. 1c . Typical results of the simulations are shown in Fig. 2 and are further discussed in the Methods. A compilation of the results of many simulations, shown in Fig. 3 , yields an approximately linear relation, Q = s ‹ z › Δ , between Q and ‹ z › Δ , where the sensitivity s =−(3.31±0.04) × 10 −9 mm −1 . From this we find Q =(−1.3±1.1) × 10 −8 ; the error here is one s.d. and derives from the statistical uncertainty in ‹ z › Δ , and does not yet include systematic effects or the ±0.04 × 10 −9 mm −1 error in the sensitivity. 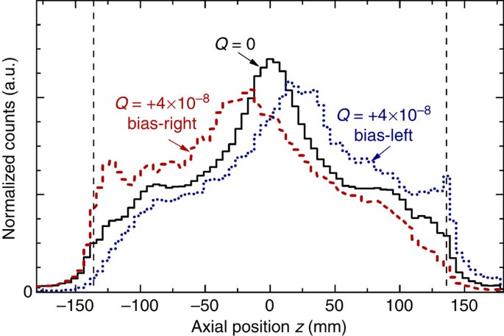Figure 2: Simulated annihilationz-distributions. Three simulated annihilationz-distributions, for antiatoms withQ=0 (black solid line) andQ=+4 × 10−8under Bias-Right (red dashed line) and Bias-Left (blue dotted line) conditions. The vertical dashed lines indicate the locations of the cuts atz= ±136 mm. Figure 2: Simulated annihilation z -distributions. Three simulated annihilation z -distributions, for antiatoms with Q =0 (black solid line) and Q =+4 × 10 −8 under Bias-Right (red dashed line) and Bias-Left (blue dotted line) conditions. The vertical dashed lines indicate the locations of the cuts at z = ±136 mm. 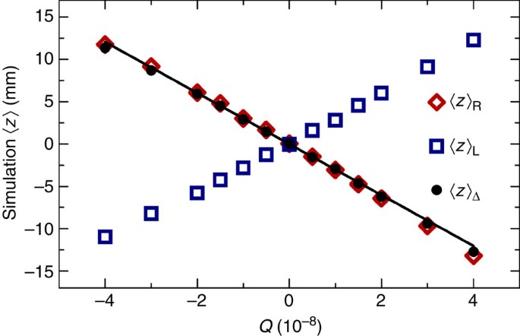Figure 3: Simulated dependence of the axial shifts onQ. The average annihilation locations ‹z› in the Bias-Right (red diamonds) and Bias-Left (blue squares) configurations, as well as the resulting ‹z›Δ(black dots), as found in the simulations with detector efficiency and resolution corrections. The statistical error of ±0.1 mm in the calculated values of ‹z›Rand ‹z›L, and ±0.07 mm for ‹z›Δ, is too small to be shown with clarity. The black solid line is the least-squares linear fit that best describes the variation of ‹z›ΔwithQ. The fit is constrained to pass through ‹z›Δ=0 atQ=0, consistent with the simulations to within statistical uncertainty and with our expectation that the bias electric fields have no effect on particles for whichQ=0. Full size image Figure 3: Simulated dependence of the axial shifts on Q . The average annihilation locations ‹ z › in the Bias-Right (red diamonds) and Bias-Left (blue squares) configurations, as well as the resulting ‹ z › Δ (black dots), as found in the simulations with detector efficiency and resolution corrections. The statistical error of ±0.1 mm in the calculated values of ‹ z › R and ‹ z › L , and ±0.07 mm for ‹ z › Δ , is too small to be shown with clarity. The black solid line is the least-squares linear fit that best describes the variation of ‹ z › Δ with Q . The fit is constrained to pass through ‹ z › Δ =0 at Q =0, consistent with the simulations to within statistical uncertainty and with our expectation that the bias electric fields have no effect on particles for which Q =0. Full size image Principle data set The annihilation location data used here were collected during experiments primarily intended to trap [4] and hold [5] antihydrogen atoms, and to eventually measure [8] the microwave spectral properties of these atoms. Thus, this analysis is a retrospective analysis of data taken for other purposes, and the data were not collected in the optimal manner for this analysis. In particular, the Bias-Right and Bias-Left conditions were not well alternated, and the antiatom synthesis sequences were varied and improved. All of the Bias-Left data were collected in 2010, and the Bias-Right data were split between 2010 (27 events) and 2011 (214 events). As our analysis relies on subtracting the means of the Bias-Right and Bias-Left data, it is critical that the experiment has not drifted in any way that could affect these means. Because of the retrospective nature of the analysis, we were limited to employing numerical simulations to analyse the potential drift mechanisms. From an extensive set of these simulations, described in the Methods, we conclude that the known systematic errors contribute an uncertainty to Q of ±0.4 × 10 −8 . By searching for a deflection of antiatoms in an electric field, we have determined that the charge Qe of the antihydrogen atom is Q =(−1.3±1.1±0.4) × 10 −8 , with a statistical confidence level of 1 σ , and close to the prediction of zero from CPT and from quantum anomaly cancellation. The only previous direct bound on the antihydrogen charge, | Q |<0.02, was deduced [18] from the observation that Q v × B forces were insufficient to deflect an energetic (momentum 1.94 GeV c −1 ) beam [26] of antihydrogen atoms away from a detector. Thus, our bound is 10 6 times more precise than the only previous direct bound. An indirect bound on the antihydrogen charge can be inferred by comparing the experimentally measured charges of the antiproton and positron. The charge anomaly of the antiproton, , is known [27] , [28] , [29] to be <7 × 10 −10 with a confidence level of 90% by measurements [28] on . The charge anomaly of the positron [27] , [31] is less well known: |( q − e )/ e |<2.5 × 10 −8 (no confidence level given explicitly, but assumed here to be 1 σ ), determined by measurements of the positron cyclotron frequency and the positronium Rydberg constant [32] . From these limits on the individual charge anomalies, we can then infer a bound on the charge of antihydrogen of | Q |<2.5 × 10 −8 . (This inference relies on the assumption that the positron and antiproton charges add exactly to form the charge of the antihydrogen atom. A similar inference was used to bound the charge anomaly of the antimuon to (−1.1±2.1) × 10 −9 by measurements of the muonium 1 s −2 s energy interval [33] .) Thus, our direct bound is ~2 times lower than the best inferred bound. It should be possible to laser cool the trapped antihydrogen atoms [34] to 20 mK. This would allow us to decrease the confining magnetic fields to make a well that is 30 mK deep, much less than the current depth of 540 mK, while still retaining the majority of the trapped antihydrogen atoms. The β in equation (3) for a 30 mK well would be lower than the current β by a factor of ~10, and the resulting bound on Q would improve by a similar factor. It would still require, however, a substantial data set. A different technique, based on stochastic acceleration [35] , [36] , could be used to bound | Q | at the 10 −12 level with only a few tens of antiatoms. Stochastic acceleration, as applied here, uses many cycles of a randomly oscillating electric field to cause antiatoms to diffuse out of the trap were they to possess a charge (see ref. 35 for details). A few cycles of oscillating electric fields were incidentally applied to the current data set. Stochastic acceleration analysis of the effect of these fields yields a bound of | Q |<2 × 10 −7 . This is roughly 10 times less precise than the deflection-based bound reported here, but more cycles of stronger electric fields applied to a cooled antihydrogen distribution could achieve the aforementioned lower bound. We note that a charge on antihydrogen could cause a significant systematic error in a gravity measurement [37] . The conducting tubes in which gravitational experiments are likely to occur all exhibit anomalous ‘patch’ electric fields. There is considerable variation [38] in the magnitude of these patch fields depending on the geometry, surface material and surface preparation of the tubes, but fields on the order of 10 −3 V mm −1 have been suggested [37] at the centre of a 10 mm tube, with fields thousands of times higher near the tube wall. These electric fields would deflect an antihydrogen atom if it had a charge; for fields of 10 −3 V mm −1 , the gravitational force would only exceed the electrical force if the charge was less than approximately 10 −7 e ; near the wall, the charge would have to be proportionally less. Thus, our measurement of the antihydrogen charge appears to be sufficient to dismiss this systematic error for an up or down gravity measurement. For a precision measurement, the tolerable charge would depend on experimental details and would likely require a more accurate measurement than we report here, but probably not more accurate than can be achieved with stochastic acceleration. Systematic effects The discussion in this section is directed towards understanding the systematic and statistical errors that affect our determination of Q . Quantitative values for the systematic errors that we analysed are listed in Table 1 . The systematic effects can be classified into one of four categories in order of descending importance (see also Table 2 ). Table 1 Systematic errors. Full size table Table 2 Systematic error formulas. Full size table Category A: systematic effects that cause the sensitivity s , the relation between Q and ‹ z › Δ , to differ from that predicted by our nominal simulations. As an example, inaccurate knowledge of the mirror coil currents would cause this type of error. These effects are assumed to be static in time. Category B: systematic effects that change with time. These effects typically change ‹ z › Δ . A z -dependent change in the performance of the detector with time would, for example, cause this type of error. While these effects could occur continuously, we estimate their size by assuming a discontinuous change between the 2010 and 2011 antiproton seasons; thus, we assume that all of the 2010 data (all of the Bias-Left data and 11% of the Bias-Right data) were collected with one value of the parameter in question, and all of the 2011 data (the remaining 89% of the Bias-Right data) were collected with a different value. Category C: similar to Category A effects, but with the sensitivity assumed to jump discontinuously between 2010 and 2011. As these errors are necessarily less than half of the Category A errors (see Table 2 ), and the Category A errors are already small, these errors will not be further discussed. Category D: systematic effects that cause an error in ‹ z ›, but not in ‹ z › Δ . An inaccurate calculation of the detector efficiency as a function of z would cause this type of error. As these errors do not affect ‹ z › Δ , they have no effect on the bounds we set on Q . All of the systematic effects described in Table 1 and in the Methods are classified into one of these four categories. Many of these effects were investigated by comparing simulations with and without the purported systematic effect. Often, the differences between the two simulations were within the sampling errors that derive from the large, but finite, number of antihydrogen trajectories modelled in the simulations. In these cases, we deem the effect to be statistically ‘insignificant’ as we do not know whether the systematic effect has a real effect on the experiment. Fortunately, all these insignificant systematic effects would have only a small effect on Q even if they were real. Here, as elsewhere where we discuss systematic errors, we define small to mean small relative to the statistical sampling errors engendered by the limited number of antihydrogen atoms that we observed. Simulation details The simulations model the antiatom equation of motion, where r is the centre of mass position of the antiatom, and E ( r , t ) and B ( r , t ) are the position and time-dependent electric and magnetic fields. For the low field seeking antiatoms modelled here, the magnetic moment, and B are antialigned. The simulations employ a symplectic propagator. The electric field in the simulation is determined by first using COMSOL and a precise model of the trap to solve Laplace’s equation for the electrostatic potential. The potential is calculated on a dense grid that covers the trapping volume, and interpolation coefficients are found for all positions. Sets of these coefficients are found for every electrode bias voltage condition employed in the experiment. The time evolution of the potential was modelled by implementing transitions between the different bias condition coefficient sets, taking into account the programmed ramp times and the measured response times of the real electrodes. The time-dependent electric field is found from the gradient of this potential. The magnetic field in the simulation is calculated from an analytic approximation accurate to better than 2% over the trap volume [25] . The magnetic field model was checked against experiments with antiprotons [25] . Detailed descriptions of similar simulations, various benchmarking tests, and the analytic magnetic field model have been given in previous publications [9] , [25] . The simulations track each antiatom for 1 s, followed by four applications of antiproton clearing electric fields [25] , the Bias-Right or Bias-Left electric fields, and finally by the magnetic field turn off. The total simulation time is 1.19 s. This sequence closely mimics the complete time history of ~71% of the antihydrogen atoms, but does not include some of the electric field manipulations used to diagnose the positron plasmas from which the antiatoms are synthesized. As these manipulations involve electric fields weaker than the bias and clearing fields, their omission has little effect. The remaining 29% of the antihydrogen atoms (36% of the Bias-Right and 17% of the Bias-Left anti-atoms) were held for times longer than ~1 s. Simulations of atoms for 10.19 s show no significant differences with respect to those held for 1.19 s. Approximately 430,000 antiatoms were simulated for each value of Q . To mimic detector resolution effects on the data, the antiatom annihilation locations were individually shifted in z by a random amount consistent with the known [24] detector resolution function. We cross-checked the primary (symplectic) simulations against fourth order, adaptive step Runge–Kutta simulations. The latter employed a somewhat more accurate magnetic field model (up to a factor of three times more accurate in some regions of the trap) and also included the electric fields induced by the changing magnetic fields; these effects were not employed in the primary simulations for reasons of computational efficiency. The differences between the results predicted by the two types of simulations are small. We also cross-checked the primary simulations against symplectic simulations employing a simplified electric field structure; in this third simulation, all trap electrodes were assumed to have the same radius. (There is a radially inwards step in the trap radius to R Wall =16.8 mm at the trap boundaries at z = ±137.6 mm.) This causes significant electric field errors at large z , for example, about 5% at z =120 mm, but again results in only small differences in Q . In all nominal simulations, is assumed to be constant. Special simulations that allow it to vary with B , as it does slightly for one of the trapped antihydrogen states (the |c> state in ref. 8 ), show that such variations have insignificant effects. Magnetic field errors Mirror coil current errors would cause various systematic errors. The coils are driven by individual power supplies rated accurate to ±0.5%. Continuous, low precision, monitoring sets upper limits of about ±1% for deviations in the mirror currents. There are small Category A, B and D effects from both differential and common mode current deviations. The maximum tilt between the axial magnetic field and the trap axis allowed by mechanical constraints, 2 mrad, produces insignificant errors. Errors or drifts in the octupole current are likewise insignificant. External magnets are a potential source of Category B and D errors, but their effect is very small. Consider an extreme example: a 1 T solenoid, 1 m long, with a bore diameter of 0.4 m. Such a solenoid would produce a shift in ‹ z › Δ on the order of 0.06 mm if it were located 2 m away from our trap during 2011. No such external magnets are even remotely this close to our experiment. Electric field errors Experimentally, the electric field is generated by multiple high voltage amplifiers driven by high precision digital to analogue converters (DACs). Each amplifier channel is accurate to ±1% and controls one trap electrode. The electric field error from one channel is anticorrelated in adjacent electrodes. Thus, the average electric field error is much smaller the error from one individual channel. The resulting error in the sensitivity s is much less than ±1% and will not be further discussed. Initial conditions for the simulations Experimentally, antihydrogen atoms are created by collisions between antiprotons and positrons. Consequently the antiatoms are born in the volume occupied by the positron plasmas. The simulations are initiated with antiatoms born in this same volume. As a check, we also ran simulations with the antiatoms born in a volume with a radius three times greater and a length two times greater. This resulted in small, insignificant Category A, B and D errors. Previous studies have established that trapped antiatoms in the ALPHA experiment have a distribution in centre-of-mass energy that scales like below the trapping threshold [5] , [25] : that is, close to a cutoff Maxwellian distribution. These studies are based on examining the time history of escaping antiatoms and show that the experimental data are much better fit by this Maxwellian distribution than by bracketing linear or uniform energy distributions. Separate examinations of the 2010 and 2011 time history data strongly suggest that the antiatom distribution did not change between these 2 years (see Fig. 4 ). Nonetheless, we can estimate the worst case effects of deviations from Maxwellian by evaluating the consequences of using a linear or uniform distribution. The resulting errors (principally Category A), while still much smaller than the statistical error, have the largest effect on Q of all of the systematic effects studied. 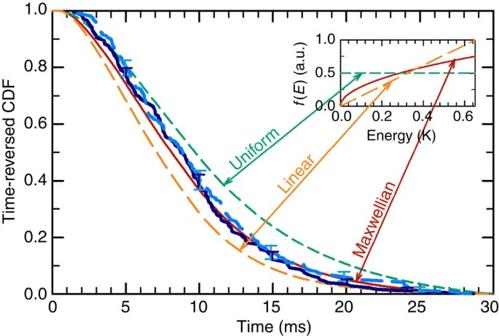Figure 4: Measured and simulated antihydrogen cumulative distribution function. The simulated time-reversed cumulative distribution function (CDF) of the time of annihilation for the nominal, Maxwellian distribution (solid red), uniform (short dashed green) distribution and linear (long dashed orange) distribution. The inset figure depicts the candidate energy distributionsf(E). The Maxwellian distribution is a much better match to both the 2010 (solid dark blue) experimental data and the 2011 (dashed light blue) experimental data than either the Uniform or Linear distributions. The error bars show the expected deviation of the CDF based on the number of observed antiatoms used to compute the CDF at each time. Figure 4: Measured and simulated antihydrogen cumulative distribution function. The simulated time-reversed cumulative distribution function (CDF) of the time of annihilation for the nominal, Maxwellian distribution (solid red), uniform (short dashed green) distribution and linear (long dashed orange) distribution. The inset figure depicts the candidate energy distributions f ( E ). The Maxwellian distribution is a much better match to both the 2010 (solid dark blue) experimental data and the 2011 (dashed light blue) experimental data than either the Uniform or Linear distributions. The error bars show the expected deviation of the CDF based on the number of observed antiatoms used to compute the CDF at each time. Full size image We have also studied anisotropic initial conditions and , where both are still consistent with the total energy distribution . (The isotropic normal condition is .) These anisotropies have a modest effect on Q . There are no obvious mechanisms that could create such anisotropies. Even if the non-cutoff distribution function were anisotropic, (a bi-Maxwellian, for instance), the cutoff, low energy portion of the distribution, from which our trapped antiatoms are sampled, would reduces to an isotropic distribution. An anisotropy would have to originate after the antiatom formation. Location errors The trap electrodes and the detector have some freedom to move relative to each other along z . We used the annihilation locations of antiprotons on background gas under poor vacuum conditions to measure this axial displacement and found that the centre of the trap is displaced from the centre of the detector by 24.0±0.2 mm. This displacement is used to shift the detector-reported locations of the antihydrogen annihilations to the electrode reference frame; thus, the 24.0 mm displacement causes no errors in our analysis (although the uncertainty of ±0.2 mm does cause a Category D error.) This displacement changed by less than ±0.34 mm between 2010 and 2011, a Category B error. The trap electrode centre could also be displaced from the magnet system centre. By employing electron cyclotron heating [39] , we have measured this displacement to be −0.5±0.5 mm. Mechanical constraints make this displacement time invariant. Detector errors The efficiency with which we can reconstruct antihydrogen annihilations is z dependent, peaking near z =0 and diminishing towards both ends. The corresponding efficiency function, Eff( z ), has been found by detailed Monte-Carlo simulations of the detector using GEANT3. It is incorporated into the simulation results by stochastically dropping simulated annihilations in a manner consistent with the efficiency function. Because of the known (and time-invariant) failure of one of the detector modules, z -asymmetries in scattering materials, and the 24.0 mm displacement between the detector and the trap centres, the efficiency is not mirror symmetric around z =0. This leads to a bias in the expected average annihilation position of ‹ z ›=0.1±3.6 mm. Fortunately, this is largely an error of Category D, which has little effect on Q . However, this also causes a small Category A error. A time-dependent variation in Eff( z ) would produce a Category B error. We have performed careful studies of the detector performance as a function of time using cosmic ray particles (typically muons) as a source; no antiparticles were present in the trap at the time of these studies. In each study, the number of ‘hits,’ and hence the ‘occupancy’, was determined for each of the 60 detector modules. (A hit is defined by the coincident detection of a signal in the orthogonally oriented detector strips on both sides of a single module, thereby allowing the location of the event that caused the signals to be determined. The occupancy is the number of particle track-forming hits per module, normalized to the number of cosmic ray events detected. The tracks were found using the standard ALPHA reconstruction methodology [24] .) From the individual occupancies, we determined the average occupancy for the modules in the right and left halves of the detector. Between 2010 and 2011 occupancies, the right occupancy changed by −0.2±0.2% and the left occupancy by 0.2±0.2%. These measurements are compatible with no change in the detector performance between the 2 years. However, we explored the consequences of these occupancies, which would lead to a real change in the detector efficiency function Eff( z ) of −0.2% on the right side and of +0.2% on the left side. As expected, this produces a small Category B error of ‹ z › Δ =−0.01±0.04 mm. We also searched for a drift in the average z -position of annihilations created during the ‘mixing’, or antihydrogen synthesis, phase of our experiment [4] , [5] , [6] , [22] . During this phase, antihydrogen atoms too energetic to be trapped, as well as re-ionized antiprotons, annihilate on the trap wall. The small observed drift is loosely equivalent to a Category B error of −0.35±0.39 mm and is statistically consistent with no detector drift. As the resolution of this technique is much poorer than that of the cosmic technique, and the results are consistent with the cosmic technique, we use the cosmic technique as our estimate of the detector error. Even if we were to use the mixing technique, however, it would be equivalent to an error in Q of only (0.13±0.15) × 10 −8 , which is significantly smaller than the sampling error. Antiproton and cosmic background Because our particle detector cannot distinguish antiprotons from antihydrogen atoms, we designed our experiment to minimize the chance that antiprotons are trapped. Measurements, comparisons with simulations and calculations have established that few, if any, antiprotons are trapped [4] , [6] , [25] ; nonetheless, it is important to estimate the magnitude of the false ‹ z › Δ signal (a Category B error) that antiprotons might engender. Previous theoretical and experimental studies of the behaviour of deliberately trapped antiprotons [25] show that all but ~5% annihilate in an elliptical region in z - t space centred on z = ±130 mm and t =5 ms, and with axial half width 20 mm and temporal half width 4 ms. Here, t =0 marks the beginning of the magnet shutdown phase of the experiment, and the sign of the z -centre is positive for Bias Right conditions and negative for Bias Left conditions (see Figures 6a and 9d in ref. 25 ). Consequently, we reduce the possible contamination from antiprotons by cutting annihilation events located within these two elliptical regions from our analysis set. To maintain symmetry, we cut with both ellipses from data taken under either Bias condition, although only one ellipse, on the appropriate side, is necessary to eliminate antiprotons from each Bias condition individually. We also cut all experimental annihilations that occur at | z |>136 mm because of the mirror maxima and the radial step in the trap wall that occurs near these locations. In addition to the z cuts, we also cut all annihilations that occur 30 ms or more after the magnet shutdown because of the increasing chance of cosmic contamination for such late events [9] . As discussed earlier, 386 events pass all cuts. (In the ~1,300 trapping trials used to obtain our event set, we would expect approximately two cosmic rays to be misclassified as antihydrogen atoms, and engender a modest error. For categorical simplicity, we list this error (and the error that comes from antiprotons) as a Category B error as these cause shifts in ‹ z › Δ ; we do not know in which year (perhaps both) the cosmic rays might have been misclassified.) A total of nine antiproton candidates are cut by the elliptical exclusion regions. It is not likely that all nine candidates are antiprotons, however, because Q =0 simulations predict that we should have observed ~7.7 antihydrogen atoms in the appropriate-side exclusion regions. Since the probability, as predicted by Poisson statistics, of observing 0 antihydrogen atoms when 7.7 are expected is P =0.0005, the likelihood that all nine candidates are antiprotons is very low. Indeed, it is not unlikely that all nine candidates are legitimate antihydrogen atoms. However, if we assume that all nine candidates are antiprotons, we would predict that an additional 9 × 0.05=0.45 antiprotons annihilate outside the exclusion regions, creating a false signal. Simulations predict that the z -averaged annihilation location of the few antiprotons outside the exclusion regions is approximately ±110 mm. Thus, for our sample size of 386 antiatoms outside of all exclusion regions, we would expect an error in |‹ z › Δ | of ~0.13 mm under the very pessimistic assumption that all nine candidates are antiprotons. Simulated z -distributions and z cuts Simulated z -distributions of antiproton annihilations are shown in Fig. 2 for antiatoms with Q =0 and for antiatoms with Q = +4 × 10 −8 under Bias-Right and Bias-Left conditions. Detector smearing and efficiency are taken into account. However, no z -cuts (that is, neither the | z |<136 mm cut nor the elliptical cut) are employed. Beyond the shifts in average z for nonzero Q , which are used to calculate ‹ z › Δ , the most remarkable feature of the data is the sharp fall-off in annihilations outside of −136 mm< z <136 mm. For Q =0, only 3.8% of the simulated particles annihilate in the outside region. (Experimentally 4.9% annihilated in the outside region. The experimental value matches the simulated value with a χ 2 P -value of 0.22.) The paucity of annihilations outside of ±136 mm is due to the location of the magnetic mirror maxima at z = ±137 mm (see Fig. 1b ) and the relative size of the axial and radial well depths. At all times after the initiation of the magnet shutdown, the axial well depth exceeds the radial well depth: for instance, at t =0 ms, it is 80 mK deeper; at t =10 ms, it is 140 mK deeper; at t =20 ms, it is 70 mK deeper; and, at t =30 ms, it is 20 mK deeper. Thus, it is always favourable for antiatoms to leave the trap radially, and few antiatoms surmount the axial well maxima. (The poor coupling [13] between the transverse and axial motions does allow a few antiatoms to escape axially.) Antiatoms with | Q |<4 × 10 −8 are also bound by the mirror maximum and largely annihilate within ±136 mm. Thus, our cut at ±136 mm is loose compared with the data, and has only a small effect on the sensitivity s . Stark forces One source of systematic error that is negligible, but deserves attention, is the Stark force that comes from polarization of the antihydrogen atoms (which we here assume is identical to that of hydrogen). The antiatoms analysed here were all held for 0.4 s or longer; this is long enough to allow for at least 99.5% of them to decay to the ground state [5] . The polarizability of ground state antihydrogen is small; given that the largest electric fields in the trap are on the order of 10 V mm −1 , and such large fields exist only in the gap between the electrodes, a value of Q greater than about 10 −14 will dominate over polarization effects. Since our bound on Q is well above this value, we can safely ignore such effects. Systematic error summary Adding all the systematic errors in Table 1 in quadrature yields a net systematic error in Q of ±0.4 × 10 −8 . As this is less than the 1 σ counting statistic error, ±1.1 × 10 −8 , the precision of our determination of Q is dominated by our sample size. Systematics also engender a net bias and error in ‹ z ›, namely 0.1±3.7 mm. Experimentally, we find an average position, ‹ z ›=3.9±3.4 mm. We stress that this bias does not enter ‹ z › Δ , and, hence, Q ; rather it provides a check on the completeness of our systematics study. Statistical methods and blind analysis The statistical techniques used here were developed using pseudo-data generated by the simulations. We investigated more complex statistical techniques than the simple averages we chose to employ, but these techniques were not found to be more powerful. We did not compute the experimental values of the averages ‹ z › R , ‹ z › L , and hence, ‹ z › Δ and Q until all of the statistical procedures were fixed and all cuts determined. The statistical Q confidence interval is based on the s.e. of the mean of the 386 event experimental data set, σ Δ z 〉 Δ =3.39±0.14 mm. We also computed the s.e. of the mean of the simulation data, assuming a 386 event subset: σ S =3.22 mm. The agreement between these two alternatives further validates the simulations and the detector efficiency curves. In principle, the sampling error of the s.e., ±0.14 mm, creates some small uncertainty in the Q confidence region range, but we do not propagate this uncertainty into the final answer. To show that our result covers zero at the 90% confidence level, we use the factor 1.64 to scale from a 1 σ confidence; Student’s t -test shows that the error in this factor due to our use of the sample rather than the population mean is negligible. Expanded data set As described above, the data analysed in this article are limited to those antiatoms that met several cut criterion in z and t , as well as to those antiatoms that were held for times greater than or equal to 0.4 s. Some likely antiatom candidates annihilated in the elliptical cut regions (designed to eliminate the possibility of including mirror-trapped antiprotons in the analysis). Others annihilated outside of | z |<136 mm. Still others were held for times between 0.17 s, the minimum hold time ever employed by ALPHA, and 0.4 s. These last antiatoms were likely to have been in the ground state, but cannot be guaranteed to have been so. Further, some antiatoms passed all cuts and were detected during trapping trials in which the Bias-Right and Bias-Left conditions were strictly alternated. As discussed earlier, most of our data were not collected in this optimal manner. In Table 3 , we compare various disjoint sets, subsets and supersets of our complete data set to our Principle data set. The Table reports ‹ z › R , ‹ z › L and ‹ z › Δ for these different data selections. The comparisons, which are summarized in Fig. 5 , show that the ‹ z › Δ are mutually consistent and are consistent with the average z annihilation position when no electric fields are applied. Table 3 Data selection. 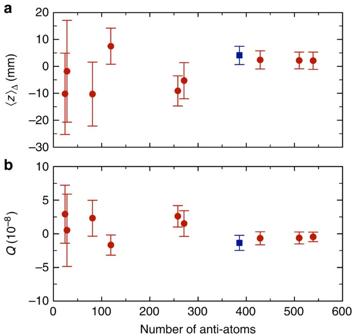Figure 5: Data selection. The ‹z›ΔandQplotted as a function of the number of antiatoms included in the analysis for the data inTable 3. The principle case is the blue square point. Note that the data are generally, but not always, cumulative with increasing number of antiatoms. Thus, the points are not generally independent. Also note that the sensitivity,s, used to scale from ‹z›ΔtoQvaries from −3.31 × 10−9mm−1(Principle data set) to −0.224 × 10−9mm−1(nozcut data sets). Ina, the error bars show the s.e. values of the mean in ‹z›Δ, and inb, these errors scaled by the sensitivitys. Full size table Figure 5: Data selection. The ‹ z › Δ and Q plotted as a function of the number of antiatoms included in the analysis for the data in Table 3 . The principle case is the blue square point. Note that the data are generally, but not always, cumulative with increasing number of antiatoms. Thus, the points are not generally independent. Also note that the sensitivity, s , used to scale from ‹ z › Δ to Q varies from −3.31 × 10 −9 mm −1 (Principle data set) to −0.224 × 10 −9 mm −1 (no z cut data sets). In a , the error bars show the s.e. values of the mean in ‹ z › Δ , and in b , these errors scaled by the sensitivity s . Full size image How to cite this article: Amole, C. et al. An experimental limit on the charge of antihydrogen. Nat. Commun. 5:3955 doi: 10.1038/ncomms4955 (2014).